Mechanistic and environmental control of the prevalence and lifetime of amyloid oligomers Amyloid fibrils are self-assembled protein aggregates implicated in a number of human diseases. Fragmentation-dominated models for the self-assembly of amyloid fibrils have had important successes in explaining the kinetics of amyloid fibril formation but predict fibril length distributions that do not match experiments. Here we resolve this inconsistency using a combination of experimental kinetic measurements and computer simulations. We provide evidence for a structural transition that occurs at a critical fibril mass concentration, or CFC, above which fragmentation of fibrils is suppressed. Our simulations predict the formation of distinct fibril length distributions above and below the CFC, which we confirm by electron microscopy. These results point to a new picture of amyloid fibril growth in which structural transitions that occur during self-assembly have strong effects on the final population of aggregate species with small, and potentially cytotoxic, oligomers dominating for long periods of time at protein concentrations below the CFC. A wide variety of peptides and proteins form self-assembled filamentous structures known as amyloid fibrils. A universal feature of all amyloid aggregates, regardless of the amino acid sequence or native conformation of the starting peptide or protein, is the formation of cross-β sheet structure [1] , [2] , [3] , [4] . Amyloid fibrils are most commonly associated with human diseases such as Alzheimer’s disease and type-2 diabetes [5] , however, they are also garnering interest in biomaterials applications [6] , [7] , [8] , [9] , [10] , [11] , [12] , [13] . Understanding the molecular mechanism(s) leading to amyloid fibril assembly is a key focus of current research. Mechanistic models of amyloid fibril self-assembly are often tested by monitoring the kinetics of formation using absorbance or fluorescence spectroscopy. The kinetics of amyloid fibril formation is typified by a lag phase followed by the onset of rapid growth. This has been attributed to the formation of a critical nucleus via primary nucleation [14] (which may be very rapid) followed by growth via fragmentation, heterogeneous nucleation or branching [15] . This classical picture has been extended to include subtle effects of protein concentration [16] , multi-stage kinetics [17] , [18] , [19] , [20] , catalytic conformational conversion [21] , [22] and competition between multiple pathways [23] . Recent research has focused on the role of fragmentation in fibril formation kinetics. Xue et al. [24] first noted that fragmentation is central to explaining the kinetics of β2-microglobulin aggregation, which cannot be described by a straightforward nucleated assembly model. More recently, analytical results show that several important features of fibril growth kinetics can be explained by a model in which fragmentation is the dominant process in fibril assembly [25] , [26] , [27] , [28] . The classical picture [29] , in which the lag time, that is, the duration of the lag phase, is determined by the formation of a thermodynamically unfavourable critical nucleus followed by fibril elongation by monomer addition, predicts that the lag time should scale with protein concentration as , where γ c =( n c +1)/2 (ref. 15 ). As the critical nucleus size n c >1, in these classical nucleation-elongation models the scaling exponent will always be greater than unity. In contrast, a model dominated by fragmentation, in which fibril fragmentation acts as a positive feedback mechanism producing new ends that can then grow, is predicted to exhibit a scaling exponent γ frag =1/2 (ref. 25 ). This prediction appears to be largely consistent with experimental observations of many known amyloidogenic protein systems. However, fragmentation-dominated models predict exponentially decaying fibril length distributions, while experimental measurements typically show distributions peaked at intermediate fibril length [30] , [31] , [32] . Here, we resolve this apparent contradiction by presenting a qualitatively new model for amyloid fibril assembly. Using a series of experiments on bovine insulin, combined with stochastic simulations, we find evidence to support the existence of a critical fibril mass concentration (CFC) above which fibrils undergo a structural transition that suppresses fragmentation. We attribute the onset of arrested fragmentation to a transition of the amyloid fibril solution from a viscous fluid to a viscoelastic gel. Our model predicts the formation of qualitatively distinct fibril length distributions for protein concentrations above and below a critical threshold and we confirm these by experiment. Moreover, we show that the concept of a structural transition that arrests the effects of fragmentation enables us to successfully predict the influence of environmental conditions on the fibril assembly pathway. Our results suggest a possible explanation for the observed variation in amyloid disease progression among apparently similar individuals: as the lengths of fibril formed depend critically on the protein concentration and are influenced by environmental conditions, in some individuals the intra- and/or inter-cellular environment may favour the formation of predominantly short and possibly toxic fibrillar species, while in other individuals conditions may result in benign fibril loads. Deviation from fragmentation-dominated models of assembly The kinetics of bovine insulin amyloid fibril formation were monitored using ThT fluorescence in 96-well microwell plates coated with a hydrophilic polymer. At least 140 replicates were performed for each set of conditions. The growth rate, k gr , and the lag time, τ lag , were extracted from the kinetic traces, averaged over replicates (as illustrated in Supplementary Fig. S1 ). Previous reports have shown the lag times measured for identical protein samples to vary by as much as hours and this has been attributed to the stochastic nature of the nucleation process [33] , [34] : in our experiments, due to careful control of experimental conditions, the variation in the lag time has been reduced to minutes ( Supplementary Fig. S2 shows individual kinetic curves for a typical experiment). Our method thus enables us to identify subtle changes in insulin amyloid fibril growth kinetics upon changing the experimental parameters. 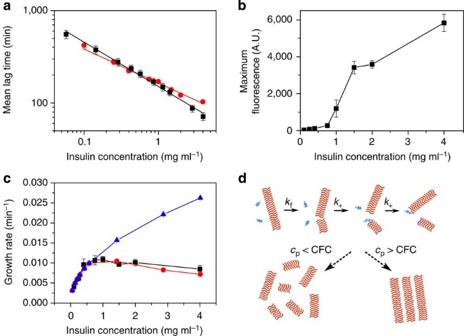Figure 1: A fragmentation model incorporating a structural transition fits kinetic data for insulin fibril assembly. (a) Lag time as a function of protein concentration. The experimental data (black squares) are fitted to the functiony=Axγwith an exponentγ=−0.37±0.02. The simulation data (red circles) have exponentγ=−0.42±0.001,k+=5 × 104M−1s−1andkf=3 × 10−8s−1. (b) Mean maximal ThT fluorescence as a function of insulin concentration. (c) Growth rate,kgr, is plotted as a function of insulin concentration. The experimental data (black squares) were obtained from kinetic curves normalized to the fluorescence maxima. The simulation data were obtained from 150 simulations per concentration using a simple fragmentation-dominated model (blue triangles), including suppression of fragmentation once the fibril mass reaches a CFC of 0.4 mg ml−1(red circles). All data points show mean±s.d. (d) In our model, fibrils grow via two processes: fragmentation, and elongation via monomer addition. These processes are characterized by their respective rateskfandk+. Our model predicts distinct fibril length distributions for protein concentrations,cpgreater or less thancT≈2CFC. Figure 1a shows how τ lag scales with the insulin concentration: the scaling exponent, γ =−0.37±0.02. As γ <1, the data are broadly consistent with a model dominated by fragmentation [25] . However, other features of our kinetic data cannot be explained by existing models. For example, the mean maximal fluorescence, that is, fluorescence at long times, rises sharply between 0.75 and 1.5 mg ml −1 insulin—an effect that is not predicted by fragmentation-dominated models ( Fig. 1b ). This effect is not caused by a change in the total fibril mass; pelleting the aggregated material by centrifugation and measuring the remaining protein in the supernatant by UV–vis spectroscopy confirmed that >99% of the total insulin present is in the pellet regardless of the initial protein concentration. Instead, we attribute the sudden order-of-magnitude increase in fluorescence to structural or morphological differences (presumably affecting the binding of the fluorophore) between fibrils formed at ‘high’ and ‘low’ insulin concentrations. It is known that the structural characteristics of amyloid fibrils are important in the binding of ThT [35] , [36] , [37] . For example, it has been shown that glucagon fibrils formed at ‘high’ (>1 mg ml −1 ) and ‘low’ (<1 mg ml −1 ) protein concentrations demonstrate markedly different structural characteristics and ThT fluorescence emission signals [38] . We measured circular dichroism (CD) spectra of insulin amyloid fibrils prepared at concentrations between 0.25 and 4 mg ml −1 and found that the spectra of the fibrils prepared at high (1–4 mg ml −1 ) and low (0.25–0.75 mg ml −1 ) protein concentrations are qualitatively different ( Supplementary Fig. S3 ). Indeed, we observed a striking transition in the CD signal between 0.75 and 1.5 mg ml −1 , consistent with the transition seen in our fluorescence measurements ( Fig. 1b ). Figure 1: A fragmentation model incorporating a structural transition fits kinetic data for insulin fibril assembly. ( a ) Lag time as a function of protein concentration. The experimental data (black squares) are fitted to the function y = Ax γ with an exponent γ =−0.37±0.02. The simulation data (red circles) have exponent γ =−0.42±0.001, k + =5 × 10 4 M −1 s −1 and k f =3 × 10 −8 s −1 . ( b ) Mean maximal ThT fluorescence as a function of insulin concentration. ( c ) Growth rate, k gr , is plotted as a function of insulin concentration. The experimental data (black squares) were obtained from kinetic curves normalized to the fluorescence maxima. The simulation data were obtained from 150 simulations per concentration using a simple fragmentation-dominated model (blue triangles), including suppression of fragmentation once the fibril mass reaches a CFC of 0.4 mg ml −1 (red circles). All data points show mean±s.d. ( d ) In our model, fibrils grow via two processes: fragmentation, and elongation via monomer addition. These processes are characterized by their respective rates k f and k + . Our model predicts distinct fibril length distributions for protein concentrations, c p greater or less than c T ≈2CFC. Full size image To better understand the nature of this transition we performed bead tracking microrheology on amyloid fibril samples at a range of insulin concentrations. We find a transition from a viscous fluid to a gel state for fibrils formed at protein concentrations above 0.75 mg ml −1 ( Supplementary Fig. S4 ). We propose that in these high concentration samples fragmentation is arrested due to the formation of a gel-like network of fibrils. Taken together, these findings lead us to propose that there exists some critical fibril mass concentration (CFC), above which fragmentation is suppressed, and that for insulin this becomes manifest in our kinetic data at protein concentrations at or above a threshold c T ∼ 0.75 mg ml −1 (see Fig. 1d ). Kinetic simulations suggest a structural transition To investigate the effects of such a structural transition on the kinetics of amyloid fibril formation and on the resulting fibril length distributions, we performed stochastic simulations of a fragmentation-dominated model of fibril growth. We first simulated a model with fragmentation and elongation only. The kinetic parameters used in the simulations were obtained by fitting our experimental data at low protein concentrations to analytical results derived by Knowles et al. [25] This resulted in fibril elongation and fragmentation rates of 5 × 10 4 M −1 s −1 and 3 × 10 −8 s −1 , respectively, (for details see Methods) and these parameters were used to generate predicted kinetic curves for a range of protein concentrations. These results were compared with our experimental data in which we normalized the growth curves to their maximal values (to decouple the growth rate measurements from the change in maximal fluorescence) and extracted the maximal growth rate, k gr ( Fig. 1c ). For low protein concentrations, we find that the values of k gr predicted by our simulations are in good agreement with our experiments. For protein concentrations above 0.75 mg ml −1 , however, our simulations of the fragmentation-dominated model fail to match our experimental results (blue curve in Fig. 1c ). To test our hypothesis that a structural transition is involved we modified our simulations so that fragmentation is arrested when the total fibril mass concentration exceeds a critical value (the CFC). Using a value for the CFC of 0.4 mg ml −1 , our simulations with fragmentation arrest reproduce our experimental results for k gr very well over the entire protein concentration range. The protein concentration c T at which the effects of the structural transition become apparent in our simulations is also in good agreement with our experimental results: c T ≈0.75 mg ml −1 . Indeed, we would expect that the CFC≈ c T /2, as for the structural transition to have any effect on the maximal growth rate k gr , it must happen before the maximal growth rate is reached, which occurs when at most half the total protein has aggregated. Figure 1a shows the simulated lag times as a function of protein concentration for comparison with experiment; our simulations incorporating the CFC give a scaling exponent of −0.42±0.001, in reasonable agreement with the experimental results. It should be noted that the precise nature of the cutoff that suppresses fragmentation in our simulations has little effect on these results ( Supplementary Fig. S5 ). Experimental length distributions match predictions Our simulations further predict, in the long-time limit, qualitatively distinct fibril length distributions for initial protein concentrations above and below the critical threshold c T . For initial protein concentrations less than c T , fibrils continue to fragment throughout the simulation, and in the long-time limit our simulations predict that the fibril length distribution will be exponential and dominated by short fibrils ( Fig. 2a ). In contrast, when the initial protein concentration is greater than c T , the mass concentration of fibrils exceeds the CFC at some time during the exponential growth phase so that fragmentation ceases. At timepoints after the CFC is reached, the fibrils still grow by monomer addition but the shape of the length distribution is fixed. This results in a log-normal fibril length distribution with a clear peak even at long times ( Fig. 2c ), in agreement with published experimental observations [30] , [31] , [32] . Supplementary Figures S6, S7 show simulated length distributions for the two regimes ( c p < c T and c p ≥ c T ) at different times during the protein aggregation kinetics. We note that fragmentation-dominated models also predict peaked distributions, but only at very early times ( Supplementary Fig. S6 ); in our model incorporating the CFC, fragmentation arrest causes these to persist. 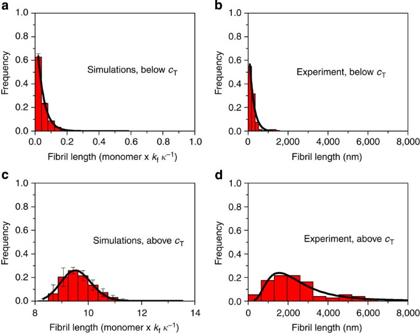Figure 2: Length distributions obtained from simulation and experiment. Fibril length distributions obtained by simulation (a) belowcT(0.2 mg ml−1) and (c) abovecT(4 mg ml−1). We express the fibril length in terms of the composite parameterkfκ−1. Our simulations do not make absolute predictions of fibril length because the choice of values ofk+andkfis not strongly constrained (see Methods), however the shape of the length distribution (plotted as a function of monomer units ×kfκ−1) is independent of this choice. The length distribution in (a) is best described by an exponential distribution; (c) is well-fitted by a log-normal distribution (black fit lines). Fibril length distributions extracted from TEM, (b) belowcT(0.2 mg ml−1,N=75, bars) and (d) abovecT(4 mg ml−1,N=159, bars). As predicted by the model, fibrils formed at protein concentrations below the CFC are significantly shorter (mean length of 231.5±230.4 nm) and the distribution is exponential (black curve). Length distributions abovecTshow a log-normal distribution (black curve) with a mean fibril length of 2,441.5±1,590.3 nm (mean±s.d.). Figure 2: Length distributions obtained from simulation and experiment. Fibril length distributions obtained by simulation ( a ) below c T (0.2 mg ml −1 ) and ( c ) above c T (4 mg ml −1 ). We express the fibril length in terms of the composite parameter k f κ −1 . Our simulations do not make absolute predictions of fibril length because the choice of values of k + and k f is not strongly constrained (see Methods), however the shape of the length distribution (plotted as a function of monomer units × k f κ −1 ) is independent of this choice. The length distribution in ( a ) is best described by an exponential distribution; ( c ) is well-fitted by a log-normal distribution (black fit lines). Fibril length distributions extracted from TEM, ( b ) below c T (0.2 mg ml −1 , N =75, bars) and ( d ) above c T (4 mg ml −1 , N =159, bars). As predicted by the model, fibrils formed at protein concentrations below the CFC are significantly shorter (mean length of 231.5±230.4 nm) and the distribution is exponential (black curve). Length distributions above c T show a log-normal distribution (black curve) with a mean fibril length of 2,441.5±1,590.3 nm (mean±s.d.). Full size image To test these predictions we used transmission electron microscopy (TEM) to obtain length distributions for amyloid fibrils formed at initial protein concentrations above and below our predicted c T of 0.75 mg ml −1 ( Fig. 2b ; see Supplementary Fig. S8 for examples of TEM images). Our experimental results are in close correspondence with our simulation predictions: we observe an exponential distribution of fibril lengths when the protein concentration is below c T and a peaked distribution, even at long times, for protein concentration above c T ( Fig. 2a ). Other studies have also reported peaked fibril length distributions [30] , [31] , [32] . We hypothesize that a structural transition may also be operating in these systems, and that these experiments may have been carried out in the high protein concentration regime where c p > c T . Adding salt enhances fibril elongation and shifts the CFC Our model further allows us to rationalize non-trivial changes in the kinetic curves when the environmental conditions are altered. It is well known that the addition of salt screens electrostatic charge, thereby decreasing the Debye length and influencing protein–protein interactions [39] . As a model environmental perturbation, we therefore repeated our kinetic experiments in the presence of increasing concentrations of NaCl. 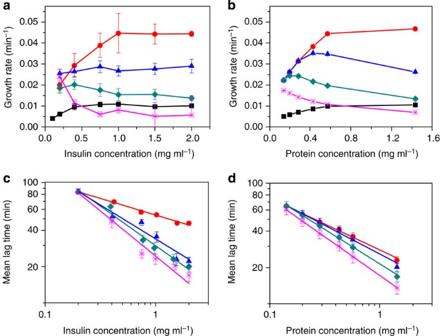Figure 3: A model incorporating a structural transition explains the effects of NaCl on aggregation kinetics. (a) Experimentalkgras a function of insulin concentration obtained from normalized traces at NaCl concentrations of 0 M (black squares), 0.1 M (red circles), 0.24 M (blue triangles), 0.34 M (dark cyan diamonds) and 0.49 M (pink stars). (b) Simulated data obtained by varying the elongation rate and the threshold for fragmentation cutoff. Parameters used in the simulations were CFC=0.4 mg ml−1,k+=5 × 104M−1s−1(black squares); CFC=0.4 mg ml−1,k+=106M−1s−1(red circles); CFC=0.2 mg ml−1,k+=106M−1s−1(blue triangles); CFC=0.1 mg ml−1,k+=106M−1s−1(dark cyan diamonds); and CFC=0.05 mg ml−1,k+=106M−1s−1(pink stars). For all simulationskf=3 × 10−8s−1. (c)τlagas a function of insulin concentration. The data are fit with same function as Fig. 1(a) resulting in scaling exponents ofγ=−0.27±0.01 (0.1 M NaCl, circles),γ=−0.56±0.05 (0.24 M NaCl, triangles),γ=−0.65±0.04 (0.34 M NaCl, diamonds),γ=−0.75±0.06 (0.49 M NaCl, stars). (d) τlagas a function of protein concentration obtained from simulations employingk+=106M−1s−1andkf=3 × 10−8s−1. The scaling exponents are −0.43±0.01 (circles), −0.47±0.02 (triangles), −0.57±0.01 (diamonds), and −0.64±0.01 (stars) when the CFC is 0.4, 0.2, 0.1 and 0.05 mg ml−1, respectively. Experimental and simulation data points show mean±s.d. Figure 3a shows k gr as a function of insulin concentration for a range of NaCl concentrations. It is clear that adding NaCl results in complicated and non-monotonic trends in the kinetics of fibril growth. In the absence of salt, our data are not dissimilar to those previously attributed to a catalytic conformational conversion at the growing end of the fibrils [21] , [22] ; the addition of salt, however, results in qualitatively and significantly different behaviour. Although these trends are not readily captured by variation of the parameters in fragmentation-dominated models, our simulations in which a structural transition is included are in good agreement with the data if we make the simple assumption that salt affects both the elongation rate ( k + in equation 1) and the CFC, but not the fragmentation rate. Such a change in the CFC is supported by our experimental data; the transition in the ThT fluorescence (as a function of protein concentration) that we plot in Fig. 1b in the absence of salt, shifts to lower insulin concentrations as the NaCl concentration is increased ( Supplementary Fig. S9 ). The results of our simulations are shown in Fig. 3b . Firstly, the increase in growth rates between 0 and 0.1 M NaCl is consistent with a ∼ 20-fold enhancement of the fibril elongation rate to 10 6 M −1 s −1 . Secondly, we capture the complex, salt-dependent and non-monotonic trends of the growth rate with protein concentration in Fig. 3a by allowing the CFC to decrease with salt concentrations above 0.1 M. It should be emphasized that the changes in the simulated curves at 0.25–0.5 M NaCl arise only from a change in the CFC; the elongation rate is held constant at 10 6 M −1 s −1 . We note that this elongation rate is subdiffusive, consistent with a requirement for some form of conformational change at the growing fibril end before the addition of each new monomer [21] , [22] , [25] . Further increasing the elongation rate does not account for the complex behaviour observed in Fig. 3a ; the presence of a structural transition in the model is essential in order to explain the experimental data. Figure 3: A model incorporating a structural transition explains the effects of NaCl on aggregation kinetics. ( a ) Experimental k gr as a function of insulin concentration obtained from normalized traces at NaCl concentrations of 0 M (black squares), 0.1 M (red circles), 0.24 M (blue triangles), 0.34 M (dark cyan diamonds) and 0.49 M (pink stars). ( b ) Simulated data obtained by varying the elongation rate and the threshold for fragmentation cutoff. Parameters used in the simulations were CFC=0.4 mg ml −1 , k + =5 × 10 4 M −1 s −1 (black squares); CFC=0.4 mg ml −1 , k + =10 6 M −1 s −1 (red circles); CFC=0.2 mg ml −1 , k + =10 6 M −1 s −1 (blue triangles); CFC=0.1 mg ml −1 , k + =10 6 M −1 s −1 (dark cyan diamonds); and CFC=0.05 mg ml −1 , k + =10 6 M −1 s −1 (pink stars). For all simulations k f =3 × 10 −8 s −1 . ( c ) τ lag as a function of insulin concentration. The data are fit with same function as Fig. 1(a) resulting in scaling exponents of γ =−0.27±0.01 (0.1 M NaCl, circles), γ =−0.56±0.05 (0.24 M NaCl, triangles), γ =−0.65±0.04 (0.34 M NaCl, diamonds), γ =−0.75±0.06 (0.49 M NaCl, stars). ( d ) τ lag as a function of protein concentration obtained from simulations employing k + =10 6 M −1 s −1 and k f =3 × 10 −8 s −1 . The scaling exponents are −0.43±0.01 (circles), −0.47±0.02 (triangles), −0.57±0.01 (diamonds), and −0.64±0.01 (stars) when the CFC is 0.4, 0.2, 0.1 and 0.05 mg ml −1 , respectively. Experimental and simulation data points show mean±s.d. Full size image Our structural transition model also helps us to understand how the lag time, τ lag , varies with salt concentration. The results of both simulation and experiment ( Fig. 3c ) show that as the salt concentration increases, the lag time becomes more protein concentration-dependent. This makes sense as our simulations indicate that adding salt has the two-fold effect of increasing the elongation rate and shifting the CFC to lower values, so that at high salt concentrations τ lag is dominated by the concentration-dependent process of fibril elongation rather than the concentration-independent process of fragmentation. The model predicts effects of adding salt during assembly If our model correctly represents the molecular mechanism of fibril assembly, then it should be able to predict what happens when the conditions are changed during the process of fibril growth. In the absence of a structural transition, we would expect that adding salt at any time before the point of maximal growth is reached will have a dramatic effect on the kinetics of fibril assembly. This is because adding salt increases the fibril elongation rate, which has a major role in determining the growth rate in fragmentation-dominated models. Plotting the growth rate as a function of the time salt is added, we would therefore expect to obtain results that follow the dashed line in Fig. 4 . However, in a model with a structural transition, salt should not influence the kinetics if it is added after the structural transition has happened—that is, after the fibril mass has exceeded the CFC. We would therefore expect to obtain the red line in Fig. 4 . Indeed, this prediction is realized in our experiments. Based on our simulation results, we predict that the CFC for the 0.3 M salt concentration used in these experiments is 0.1 mg ml −1 , and that the CFC should be reached at ∼ 110 min. Indeed, we find that adding NaCl at any time before the predicted CFC is reached (that is, before 110 min) results in a strong increase in k gr , but after 110 min, adding salt has no effect—that is, our experiments indeed follow the red line rather than the dashed line in Fig. 4 . 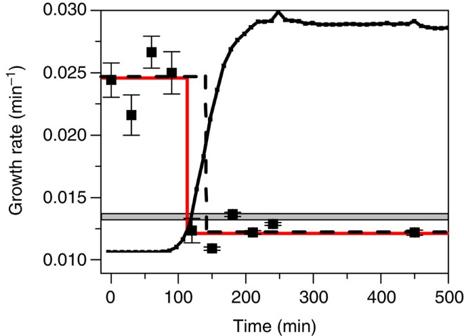Figure 4: The influence of environment on the growth kinetics. A series of 1.5 mg ml−1insulin samples were incubated simultaneously. At specific time points during the kinetics of self-assembly (every 30 min), NaCl was added to three samples. The mean value ofkgrfrom the resulting kinetic traces of each group of samples is plotted against the time at which the NaCl was added (squares). To illustrate where on the kinetic profile the NaCl was added, the kinetic trace for the control is also shown (triangles). The grey box corresponds to the meankgr±s.d. for this salt-free control. In the absence of any structural transition, we would expect to observe the behaviour shown by the dashed line, with enhanced growth rates during the early stages of fibril assembly, returning to control values if salt is added after the point at whichkgris measured (∼160 min). With the existence of a CFC, we would expect instead the trend inkgras shown by the solid line; the decrease inkgrnow occurs the moment the CFC is reached. Indeed, we observe thatkgrdecreases to the control value when salt is added at any time after 120 min, consistent with the sample having reached the CFC, which for 1.5 mg ml−1insulin under these conditions we estimate to occur at 110 min. Figure 4: The influence of environment on the growth kinetics. A series of 1.5 mg ml −1 insulin samples were incubated simultaneously. At specific time points during the kinetics of self-assembly (every 30 min), NaCl was added to three samples. The mean value of k gr from the resulting kinetic traces of each group of samples is plotted against the time at which the NaCl was added (squares). To illustrate where on the kinetic profile the NaCl was added, the kinetic trace for the control is also shown (triangles). The grey box corresponds to the mean k gr ±s.d. for this salt-free control. In the absence of any structural transition, we would expect to observe the behaviour shown by the dashed line, with enhanced growth rates during the early stages of fibril assembly, returning to control values if salt is added after the point at which k gr is measured ( ∼ 160 min). With the existence of a CFC, we would expect instead the trend in k gr as shown by the solid line; the decrease in k gr now occurs the moment the CFC is reached. Indeed, we observe that k gr decreases to the control value when salt is added at any time after 120 min, consistent with the sample having reached the CFC, which for 1.5 mg ml −1 insulin under these conditions we estimate to occur at 110 min. Full size image Prevalence of small molecular weight species Small molecular weight species, including short fibrils, that are present during the assembly of amyloid fibrils are of particular interest because they are thought to be the causative agents of toxicity [40] , [41] , [42] , [43] . Our model makes a strong prediction that the prevalence of short fibrils should be very different for protein concentrations above and below the critical threshold. 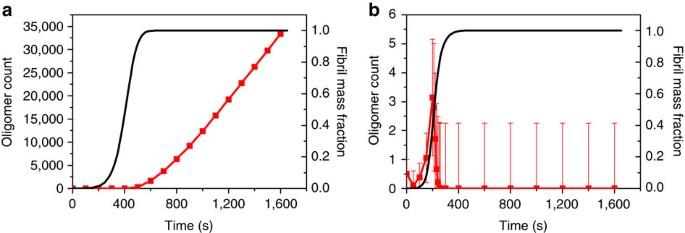Figure 5: Oligomer populations as a function of time. The number of short fibrils, of ≤100 monomer units, plotted as a function of time (red squares); kinetic traces of the total fibril mass (normalized, right axes) are also shown (black lines). (a) Atcp=0.2 mg ml−1, the protein concentration is belowcTand a large number of short fibrillar species persist for long periods of time. (b) Atcp=0.85 mg ml−1, a maximum in short species occurs at a time approximately coincident with the CFC being reached. Once the CFC is reached and the structural transition takes place, this population diminishes due to the suppression of fragmentation. The data are derived from stochastic simulations and are shown as the mean±s.d. of 150 replicate runs. Figure 5a shows the prevalence of short fibril species in our simulations as a function of time. For c p > c T , we predict the transient formation of a small population of short fibrils, peaking approximately half-way through the growth phase before returning to low levels ( Fig. 5b ). When c p < c T , however, the number of short fibrils is predicted to be much greater and increasing with time ( Fig. 5a ). Thus, the structural transition has a dramatic influence on the prevalence of potentially cytotoxic species during amyloid fibril assembly. Figure 5: Oligomer populations as a function of time. The number of short fibrils, of ≤100 monomer units, plotted as a function of time (red squares); kinetic traces of the total fibril mass (normalized, right axes) are also shown (black lines). ( a ) At c p =0.2 mg ml −1 , the protein concentration is below c T and a large number of short fibrillar species persist for long periods of time. ( b ) At c p =0.85 mg ml −1 , a maximum in short species occurs at a time approximately coincident with the CFC being reached. Once the CFC is reached and the structural transition takes place, this population diminishes due to the suppression of fragmentation. The data are derived from stochastic simulations and are shown as the mean±s.d. of 150 replicate runs. Full size image The key finding in this study is the identification of a CFC above which insulin amyloid fibrils undergo a structural transition that suppresses fragmentation. Using a very simple model that includes this feature we are able to successfully simulate the complex behaviour that we observe in our kinetic experiments under a variety of solution conditions. Indeed, the shapes of the length distributions we found from simulation and TEM experiments for fibrils formed above the critical concentration are similar to those found in previous experiments [30] , [31] , [32] , although both simulations and our TEM experiments show very different, exponential-like length distributions at protein concentrations below the predicted structural transition. It has become the general consensus that small oligomeric aggregates are the causative agents of cytotoxicity [40] , [41] , [42] , [43] , [44] , whereas the mature, long fibrils are the inert end product of assembly [45] , [46] . Importantly, Xue and co-workers [47] have demonstrated that it is not just the oligomers formed during self-assembly that are toxic, but that short fibrils generated through the fragmentation of mature fibrils also cause cell death. Intriguingly, multiple studies have shown that there is no direct correlation between fibril load within tissue (that is, mass of long fibrillar material) and loss of function [45] , [46] , [48] , [49] , [50] , [51] , [52] , [53] . Indeed, it has been shown that a significant fraction of members of the Nun study [54] possessed neuritic β-amyloid plaques and neurofibrillary tangles at the time of death without exhibiting any cognitive dysfunction. The observation that in some cases fibrils can be present but not cause measurable functional impairment could be due to amyloid fibril assembly pathways that favour the rapid formation of longer inert fibrils as a result of the local intracellular environment. Our observation of two distinct length distributions that are determined only by the environmental conditions, one of which is comprised of long, potentially inert fibrils microns in length while the other is dominated by very short, possibly toxic, fibrillar species, may have consequences for determining the propensity of intracellular conditions to bias toward either benign or cytotoxic fibrillar loads. To this end, we have shown that salt concentration has a strong impact on the value of the CFC. Higher salt concentrations shift the CFC to lower values, stabilizing the length distribution for lower initial concentrations of protein. In our study, we chose salt as a tool to alter protein–protein and fibril–fibril interactions, but any additive or solution condition that can affect the charge characteristics or protein structure, such as pH, temperature or the presence of hydrophobic surfaces, could affect the value of CFC. This could have far-reaching consequences for toxicity in intracellular environments, where salt gradients, pH differences, the presence of chaperones and other co-factors could bias toward the formation of toxic or non-toxic fibrillar species. Interestingly, Taylor et al. [55] map the level of Aβ(1–40) cytotoxicity to the kinetic profile of fibril formation, reporting a peak in cytotoxicity during the exponential growth phase of assembly. After this peak is reached, cytotoxicity decays back to baseline levels at the point in the kinetic profile where fibril assembly approaches and reaches the final plateau. The results of Taylor et al. [55] may be interpreted in the context of our structural transition model: a population of small molecular weight species is generated through fragmentation, and then depleted by the combined influence of fragmentation inhibition owing to a structural transition and fibril elongation. Applying our model to the data presented in [55] we would predict the CFC for Aβ(1–40) to be ∼ 0.15 mg ml −1 ( ∼ 35 μM). In our simulations at high protein concentrations, the presence of short, potentially cytotoxic oligomeric species shows very similar kinetics to the kinetics of cytotoxicity reported by Taylor et al. ( Fig. 5b ). For simulations in which the initial protein concentration is above c T , we find an analogous peak in small molecular weight species mid-way through the exponential growth phase, which is followed by a decay back to baseline levels. In contrast, when the concentration of protein is below c T , the residence time of small, potentially toxic species is significantly longer: indeed they remain present in high abundance even at very long times ( Fig. 5a ). This could have profound consequences for the propensity for cellular damage or death when intracellular conditions are such that short fibrils are the more likely species to be present. If this is indeed the case, then it may be possible to devise therapeutic measures that take advantage of these insights to alter cellular conditions so as to bias toward the accumulation of longer inert fibrils and away from the shorter toxic species. Amyloid and amyloid-like fibrils have also received attention for their potential use biomaterials or components in composite materials [13] . For example, Reches and Gazit [10] have used fibrils to template metal nanowires, Channon et al. [6] have used them as the basis for light harvesting structures and a number of authors (for example, Zhang [7] ; Zhang et al. [8] ; and Gras et al. [56] ) have used them as the basis for cell scaffolds. A significant challenge remains in controlling the length distribution of fibres, and the viscoelasticity of the resulting hydrogel. Our current findings suggest mechanisms for manipulating both, and for predicting and controlling the homogeneity of the resulting population. Insulin sample preparation Bovine insulin was obtained from Sigma-Aldrich (I5,500, lot no. 0001434060). The zinc content was ∼ 0.5% (w/w). The samples in this study were dissolved in 25 mM HCl (pH 1.6) immediately before the experiment. All solvents and solutions were filtered through a 0.22 μm filter (Millipore). Concentrations were checked via UV–vis absorption spectroscopy. ThT was added to each solution to a final concentration of 20 μM. ThT fluorescence kinetic measurements The ThT fluorescence measurements were conducted using a BMG Labtech Fluostar plate reader and Corning NBS 96-well plates (Corning 3641). Each well of the plate was filled with 100 μl of solution. Experiments for each protein concentration were replicated across 2–3 whole plates. The plates were incubated at 60 °C and fluorescence readings were taken from the bottom of the plate at wavelengths of 450 nm for excitation and 485 nm for emission. Readings were taken every 10 min. The final number of individual experiments for a given concentration ranged from 140–200. Transmission electron microscopy Samples were deposited onto 400 mesh copper grids (Taab, Aldermaston, UK) coated with formvar and carbon. Insulin solutions were incubated at 60 °C in eppendorf tubes. The 4 mg ml −1 sample was subsequently diluted 20-fold. Aliquots of 3 μl insulin fibrils were placed on the grids. After 5 min the grids were washed with 10 μl MilliQ water followed by an application 4 μl of 2% uranyl acetate (w/v). The uranyl acetate was left on the sample grid for 30 s. Excess water and stain were removed with filter paper and the grids were left to air-dry for 20 min. Imaging was performed using a Philips (FEI) CM120 Biotwin transmission electron microscope with an operating voltage of −80 kV. Fibrils lengths were determined using ImageJ image analysis software. CD spectroscopy Readings were taken using a Jasco J-810 spectropolarimeter. Samples were prepared in microwell plates as described above and then transferred to a quartz cuvette with a path length of 0.1 mm. Spectra were obtained by averaging over five accumulations. A bandwidth of 1 nm and sensitivity of 100 mdeg was used in all experiments. Bead tracking microscopy Insulin samples were incubated at 60 °C and the resulting fibril solution were placed on a glass slides. One micron beads latex beads were added and the slides sealed with a glass cover slip and petroleum jelly. Images were captured using a Nikon Ti-U inverted microscope, × 40 ELWD objective and a Mikrotron EoSens CCD camera with a capture rate of 100 fps. Subsequent images were analysed using standard particle tracking software in IDL [57] . Stochastic simulations Our simulations utilized the Gillespie algorithm [58] . Our simulation model consists of the following set of chemical reactions: Here, f i denotes a fibril of length i and m denotes a protein monomer. We assume that the shortest possible fibril length is two monomer units (that is, the ‘nucleus size’ is 2). Reaction (1) represents elongation by monomer addition, with rate constant k + (the factor of 2 arises from the fact that monomers can be added at either end of a fibril). Reaction (2) represents fragmentation of a fibril into two shorter fibrils: k f is the fragmentation rate, which we assume to be independent of the position along the fibril at which fragmentation happens. Note that this reaction also incorporates monomer loss from the fibril ends (here f 1 ≡ m ). In our simulations, we track explicitly the growth and fragmentation of individual fibrils. For reasons of computational speed, we used a system volume of 0.83 pL. We find that our simulations best fit our experimental data (in particular for the scaling of lag time with protein concentration) if they were started with a single dimer. Each simulation data point shown represents the average of 150 replicate runs, each comprising 10 5 s of simulated time. The values of k + and k f were obtained by fitting our experimental data, in the low concentration regime c p ≤ c T , to the analytical result for a simple fragmentation model, presented by Knowles et al. [59] . This provides the composite parameter from which we choose elongation and fragmentation rates, setting the fragmentation rate in accordance with our previous findings [59] ( k + =5 × 10 4 M −1 s −1 ; k f =3 × 10 −8 s −1 ). Within the constraint set by κ, the precise choice of k + and k f influences the average fibril length at long times, but does not significantly affect our predictions for the growth kinetics. Fitting to the data from experiments performed with the lowest salt concentration (0.1 M NaCl) yields k + =10 6 M −1 s −1 and k f =3 × 10 −8 s −1 . For simulations that include the structural transition, the fragmentation rate k f is switched to zero when the fibril mass concentration exceeds the CFC. We also investigated the effect of implementing a softer transition. Here, we instead scale the fragmentation rate by a factor y =(1/2)[1−tanh ( A ( F —CFC))], where the coefficient A controls the sharpness of the transition; this corresponds to the hard cutoff when A →∞. This softening of the cutoff does not result in significant changes to the kinetics. For more details see Supplementary Fig. S5 . How to cite this article: Morris, R. J. et al. Mechanistic and environmental control of the prevalence and lifetime of amyloid oligomers. Nat. Commun. 4:1891 doi: 10.1038/ncomms2909 (2013).